The rainbow trout genome provides novel insights into evolution after whole-genome duplication in vertebrates Vertebrate evolution has been shaped by several rounds of whole-genome duplications (WGDs) that are often suggested to be associated with adaptive radiations and evolutionary innovations. Due to an additional round of WGD, the rainbow trout genome offers a unique opportunity to investigate the early evolutionary fate of a duplicated vertebrate genome. Here we show that after 100 million years of evolution the two ancestral subgenomes have remained extremely collinear, despite the loss of half of the duplicated protein-coding genes, mostly through pseudogenization. In striking contrast is the fate of miRNA genes that have almost all been retained as duplicated copies. The slow and stepwise rediploidization process characterized here challenges the current hypothesis that WGD is followed by massive and rapid genomic reorganizations and gene deletions. Whole-genome duplications (WGDs) are rare but dramatic events resulting in a sudden doubling of the complete genome sequence. While WGDs are rare within animal lineages, they deeply shaped vertebrate evolution [1] and represent important evolutionary landmarks from which some major lineages have diversified. For instance, the ancestral genome of all teleost fish underwent a WGD, termed here the teleost-specific 3rd WGD (Ts3R) [2] , [3] , that has been dated 225 to 333 million years ago (Mya) [4] , [5] , [6] ( Fig. 1 ). The signature of this Ts3R is still present in modern teleost genomes [2] , [7] , [8] and was preceded by two older WGD events common to all bony vertebrates [9] . Following WGD, the resulting duplicated genomes eventually retain only a small proportion of duplicated genes, while seemingly redundant copies are inactivated by a process termed gene fractionation [10] . To date, this gene fractionation process has been poorly investigated in vertebrates because all well-characterized WGDs are extremely ancient [2] , [8] , [9] and gene fractionation is thought to be completed in these species. Salmonids are thus of particular interest in that context as gene fractionation may still be ongoing in their lineage because of an additional and relatively recent WGD event (the salmonid-specific 4th WGD or Ss4R) that has been dated 25 to 100 Mya [11] ( Fig. 1 ). Rainbow trout ( Oncorhynchus mykiss ) is a member of the salmonid family that is of major ecological interest worldwide. It is one of the most studied fish species and is extensively used for research in many fields such as carcinogenesis, toxicology, immunology, ecology, physiology and nutrition [12] . It is also an important aquaculture species of major economic importance raised in both hemispheres and on all continents. 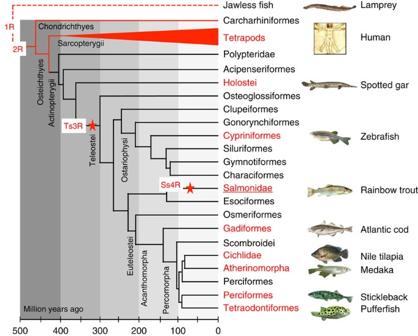Figure 1: Evolutionary position of the rainbow trout. This tree is based on the time-calibrated phylogeny information from Nearet al.4except for the additional branches in red. The red stars show the position of the teleost-specific (Ts3R) and the salmonid-specific (Ss4R) whole-genome duplications. Groups of species in which a genome sequence is available are shown in red bold type, with one example in each group. Origin of fish pictures: Manfred Schartl and Christoph Winkler (medaka, zebrafish and Tetraodon), John F. Scarola (rainbow trout), Bernd Ueberschaer (Nile tilapia) and Konrad Schmidt (three-spined stickleback). Figure 1: Evolutionary position of the rainbow trout. This tree is based on the time-calibrated phylogeny information from Near et al. [4] except for the additional branches in red. The red stars show the position of the teleost-specific (Ts3R) and the salmonid-specific (Ss4R) whole-genome duplications. Groups of species in which a genome sequence is available are shown in red bold type, with one example in each group. Origin of fish pictures: Manfred Schartl and Christoph Winkler (medaka, zebrafish and Tetraodon), John F. Scarola (rainbow trout), Bernd Ueberschaer (Nile tilapia) and Konrad Schmidt (three-spined stickleback). Full size image Due to a relatively recent WGD, the rainbow trout thus provides a unique opportunity to better understand the early steps of gene fractionation. Our results based on the analysis of the whole-genome sequence of rainbow trout show that despite 100 million years of evolution the two ancestral subgenomes have remained extremely collinear. Only half of the protein-coding genes have been retained as duplicated copies and genes have been lost mostly through pseudogenization. In striking contrast with protein-coding genes is the fate of miRNA genes that have almost all been retained as duplicated copies. Together our results reveal a slow and stepwise rediploidization process that challenges the current hypothesis that WGD is followed by massive and rapid genomic reorganizations and gene deletions. Genome structure evolution after the Ss4R WGD To obtain a global representation of the two copies of the ancestral salmonid genome in the modern rainbow trout genome, we reconstructed double-conserved synteny (DCS) regions [13] (that is, paralogous regions originating from the Ss4R). The organization of the ancestral karyotype of salmonids prior to Ss4R was reconstructed using comparisons with non-salmonid teleost genomes ( Fig. 2a ). In addition, we reconstructed the more ancient paralogy relationships inherited from the Ts3R event ( Fig. 2b , Supplementary Table 1 ). The rainbow trout genome is organized into 38 pairs of large duplicated regions distributed over the 30 chromosomes, 14 of which result from the fusion of two different post-Ss4R chromosomes, in agreement with the known paralogies inferred from the trout linkage maps [14] . Other chromosomes are more complex mosaics of different post-Ss4R chromosomes ( Fig. 2c ), reflecting additional inter-chromosomal rearrangements that have occurred since the Ss4R event ( Fig. 2d ). 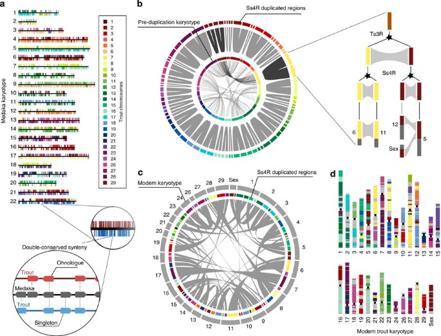Figure 2: Evolutionary history of the duplicated trout genome. (a) Double-conserved synteny between the trout and medaka genomes. Each medaka chromosome (represented as a horizontal black line) is mostly syntenic with two different chromosomes in the trout genome (syntenic trout regions represented on either side by different colours according to their chromosomal location), a pattern typically associated with whole-genome duplication. Pairs of paralogous trout genes that are inserted in a double-conserved synteny block compared to a non-salmonid fish genome are consistent with an origin at the Ss4R event (ohnologues), while genes that are inserted in a double-conserved synteny block but have no paralogue are singletons that have lost their duplicate copy since the Ss4R event. Only genes anchored to a trout chromosome are represented. (b) Successive rounds of duplication in the trout genome. The double-conserved synteny pattern between trout and non-salmonid fish delineates large chromosomal regions in the trout genome that are Ss4R duplicates of each other (outer circle, joined by grey links), descended from the same ancestral region. These ancestral pre-duplication regions could be grouped into 31 ancestral chromosomes (inner circle) based on the organization of their orthologous counterparts in non-salmonid genomes. The ancestral pre-duplication karyotype itself is an ancient tetraploid following the Ts3R event: Ts3R-duplicated regions in the pre-duplication karyotype are highlighted by grey links within the inner circle. On the right is detailed the evolutionary history of one ancestral genomic region that gave rise to paralogous regions in chromosomes 6/11 and 5/12/Sex through the Ts3R and Ss4R successive WGD events. (c) Chromosomal organization of the modern rainbow trout genome. Colours as in (b); duplicated regions are joined by grey links. Most modern trout chromosomes result from a fusion between two Ss4R-duplicated blocks descending from different ancestral chromosomes. The order of the duplicated blocks within each modern chromosome does not necessarily reflect the actual organization of the chromosome, as gene orders may have been reshuffled by intra-chromosomal rearrangements (see (d)). (d) Modern organization of the Ss4R-duplicated regions in the trout genome. Colours are as in (b,c). Figure 2: Evolutionary history of the duplicated trout genome. ( a ) Double-conserved synteny between the trout and medaka genomes. Each medaka chromosome (represented as a horizontal black line) is mostly syntenic with two different chromosomes in the trout genome (syntenic trout regions represented on either side by different colours according to their chromosomal location), a pattern typically associated with whole-genome duplication. Pairs of paralogous trout genes that are inserted in a double-conserved synteny block compared to a non-salmonid fish genome are consistent with an origin at the Ss4R event (ohnologues), while genes that are inserted in a double-conserved synteny block but have no paralogue are singletons that have lost their duplicate copy since the Ss4R event. Only genes anchored to a trout chromosome are represented. ( b ) Successive rounds of duplication in the trout genome. The double-conserved synteny pattern between trout and non-salmonid fish delineates large chromosomal regions in the trout genome that are Ss4R duplicates of each other (outer circle, joined by grey links), descended from the same ancestral region. These ancestral pre-duplication regions could be grouped into 31 ancestral chromosomes (inner circle) based on the organization of their orthologous counterparts in non-salmonid genomes. The ancestral pre-duplication karyotype itself is an ancient tetraploid following the Ts3R event: Ts3R-duplicated regions in the pre-duplication karyotype are highlighted by grey links within the inner circle. On the right is detailed the evolutionary history of one ancestral genomic region that gave rise to paralogous regions in chromosomes 6/11 and 5/12/Sex through the Ts3R and Ss4R successive WGD events. ( c ) Chromosomal organization of the modern rainbow trout genome. Colours as in ( b ); duplicated regions are joined by grey links. Most modern trout chromosomes result from a fusion between two Ss4R-duplicated blocks descending from different ancestral chromosomes. The order of the duplicated blocks within each modern chromosome does not necessarily reflect the actual organization of the chromosome, as gene orders may have been reshuffled by intra-chromosomal rearrangements (see ( d )). ( d ) Modern organization of the Ss4R-duplicated regions in the trout genome. Colours are as in ( b , c ). Full size image Timing of the Ss4R WGD We defined as ohnologues (that is, paralogues formed by a WGD event) [15] 6,733 pairs of trout-specific paralogues identified in DCS regions, and therefore consistent with an Ss4R origin. We computed the distribution of silent substitutions (dS) among pairs of Ss4R ohnologues (modal value=0.1875) and between Atlantic salmon and rainbow trout pairs of orthologues (modal value=0.055; Fig. 3a ). Based on the speciation between Salmo and Oncorhynchus genera that is dated 28.2 Mya (±1.6 Mya) [16] and assuming a constant rate of substitution, we estimated by linear extrapolation the date of the Ss4R at 96 Mya (±5.5 Mya) ( Fig. 3b ). 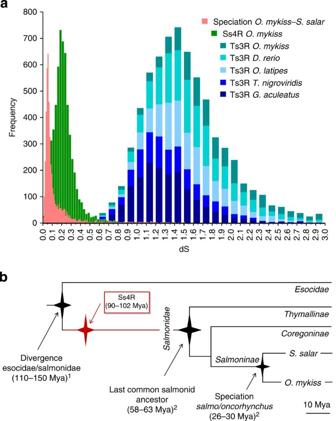Figure 3: Timing of the salmonid-specific 4th round of genome duplication (Ss4R). (a) Frequency distribution of dS values for pairs of genes in fish genomes. The distribution of dS values between Atlantic salmon and rainbow trout orthologues (pink;n=4,854) measures the neutral evolutionary divergence since the two species diverged, while values computed between trout Ss4R paralogues (green;n=6,099) measure the divergence since the more ancient Ss4R. Both events are much younger than the teleost WGD represented by within-species comparisons of paralogues (Ts3R: stickleback,n=1,671; tetraodon,n=974; medaka,n=1,393; zebrafish,n=1,717; trout,n=1,111). Note that in order to represent all the data on the same frequency scale, bin sizes are different for each data set. (b) Evolution of salmonids and the Ss4R timing. The timing of the salmonid radiation (2) and of the speciation ofSalmoandOncorhynchus(2) was based on Crête-Lafreniereet al.16, and the divergence time between Esocidae and Salmonidae (1) was based on Nearet al.4. Figure 3: Timing of the salmonid-specific 4th round of genome duplication (Ss4R). ( a ) Frequency distribution of dS values for pairs of genes in fish genomes. The distribution of dS values between Atlantic salmon and rainbow trout orthologues (pink; n =4,854) measures the neutral evolutionary divergence since the two species diverged, while values computed between trout Ss4R paralogues (green; n =6,099) measure the divergence since the more ancient Ss4R. Both events are much younger than the teleost WGD represented by within-species comparisons of paralogues (Ts3R: stickleback, n =1,671; tetraodon, n =974; medaka, n =1,393; zebrafish, n =1,717; trout, n =1,111). Note that in order to represent all the data on the same frequency scale, bin sizes are different for each data set. ( b ) Evolution of salmonids and the Ss4R timing. The timing of the salmonid radiation (2) and of the speciation of Salmo and Oncorhynchus (2) was based on Crête-Lafreniere et al. [16] , and the divergence time between Esocidae and Salmonidae (1) was based on Near et al. [4] . Full size image Gene fractionation after the Ss4R WGD To analyse gene fractionation in greater detail, we selected a subset of 569 pairs of high-confidence paralogous regions sharing at least four Ss4R ohnologous genes. These 569 DCS regions contain 13,352 genes (29% of all the protein-coding genes), which are the descendants of 9,040 pre-Ss4R ancestral genes that are now represented by 4,728 single-copy genes (singletons) and 4,312 pairs of ohnologues. Across the entire genome, this would mean that only 52% of the Ss4R duplicated gene pairs have undergone gene fractionation and returned to a single-copy state, while 48% have retained both ohnologues. Additionally, we systematically aligned protein sequences predicted from singletons to their ohnologous genomic region, and found that the majority of singletons (66%) can still be paired with clear paralogous sequences stemming from the Ss4R, although the latter are largely non-functional. In addition to the high retention rate of ohnologous protein-coding genes, we found that the post-Ss4R conservation of miRNAs genes is even more pronounced. We identified 241 miRNA loci in DCS regions of the rainbow trout genome. Among these 241 loci, 233 are present in duplicated copies (97%) while 8 loci only display one member of the ohnologous pair (3%). A ratio of 3.04 loci per mature miRNA sequence was observed in rainbow trout ( Supplementary Table 2 ). In teleosts that have undergone Ts3R WGD without the additional and more recent Ss4R WGD, the number of loci per mature miRNA ranges between 1.22 and 1.45. In vertebrate species that have not undergone Ts3R (that is, tetrapods in Supplementary Table 2 ), this ratio is close to 1 and similar to the ratio observed in non-vertebrate metazoan species in which no WGD has been reported. Mature and pre-miRNA sequences are short sequences exhibiting an average size of 22 and 70 nucleotides, respectively. These sequences are much shorter than mRNA sequences and the chance of fixing a mutation leading to pseudogenization could then be simply reduced due to these size differences. We tested this simple size hypothesis by looking at the size differences between ohnologues and singletons and the size differences within pseudogenes. We found that singleton genes are significantly smaller than genes retained as ohnologues (1,065 bp versus 1,435 bp; pval≤2.2 10 −16 ). In addition, the percentage of divergence of the pseudogenes with their functional singleton homologues is not correlated with their size ( r 2 =0.02). These two results demonstrate that, at least for protein-coding genes, longer sequences are not more prone to accumulate mutations and that this size effect is an unlikely explanation for the retention of all miRNA genes as duplicate copies in the rainbow trout genome. Gene inactivation rate after the Ss4R WGD The rainbow trout genome assembly contains 46,585 annotated protein-coding genes. Assuming that these are distributed similarly as observed on the 569 high-confidence DCS regions, they correspond to 48% of ancestral pre-WGD genes retained as ohnologues and 52% retained as singletons. As such, we estimate that the ancestral pre-WGD genome contained 31,476 genes (95% CI: 31,265–31,690), 16,368 of which have been retained as singletons in the modern trout genome (95% CI: 16,162–16,795). The second copy of these genes has been inactivated since the Ss4R WGD, leading to an average gene inactivation rate of 170 genes per million years since the Ss4R in the rainbow trout lineage (95% CI: 168–175). Colinearity of Ss4R paralogous genomic regions At the genome organization level, the analysis of the Ss4R duplicated regions reveals a high colinearity between paralogous genomic sequences, consistent with a conserved order of ohnologues (97.7% of conserved gene adjacencies) and no strong evidence of a clustering of singletons versus ohnologues throughout the genome ( Fig. 4a–c ; Supplementary Fig. 1 ). We also found that the nucleotide sequence identity between alignable paralogous genomic regions is still high (86%) and that Ss4R ohnologous protein-coding sequences and miRNAs are also highly conserved in their sequences with 92.9% amino-acid identity (SD=2.7%; Fig. 4c ) and 96.4% nucleotide identity (SD=2.9%), respectively. In addition, the identity between the Ss4R protein-coding singletons and their corresponding pseudogenes remains high (average amino-acid identity 79.0%, SD=5.5%; Fig. 4c and Supplementary Fig. 2 ). 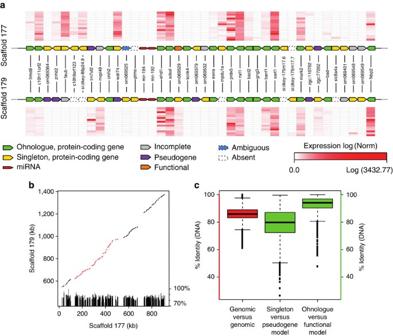Figure 4: Conserved organization of the Ss4R duplicated regions. (a) Two ohnologous scaffolds (177 and 179) are aligned, showing the perfect conservation of ohnologous gene (green) order typically found in most ohnologous scaffolds. When no onhologous copy was annotated, the singleton gene copy (yellow) was used to build a gene model when possible, leading to five possible outcomes: functional (orange), pseudogene (purple), incomplete gene model (grey), absent (that is, no match, white) or ambiguous (blue). Normalised expression values are shown for each annotated protein-coding gene for 15 tissues. (b) The plots show the result of the LastZ alignment of the genomic DNA sequence of two scaffolds. The histogram underneath indicates the local percentage of nucleotide sequence identity of each LastZ High-scoring Segment Pair (HSP). The section in red corresponds to the region shown in panel (a). (c) Whisker plots (with whiskers representing the range of the distribution, excluding the 5% most extreme values) showing the distribution of percentage of nucleotide sequence identity between LastZ HSPs of 579 ohnologous scaffolds (n=85,050, red), and the percentage of amino-acid sequence identity between single-copy genes and their pseudogene model (n=1,344, green) or ohnologous gene copies between each other (n=4,032, green). Figure 4: Conserved organization of the Ss4R duplicated regions. ( a ) Two ohnologous scaffolds (177 and 179) are aligned, showing the perfect conservation of ohnologous gene (green) order typically found in most ohnologous scaffolds. When no onhologous copy was annotated, the singleton gene copy (yellow) was used to build a gene model when possible, leading to five possible outcomes: functional (orange), pseudogene (purple), incomplete gene model (grey), absent (that is, no match, white) or ambiguous (blue). Normalised expression values are shown for each annotated protein-coding gene for 15 tissues. ( b ) The plots show the result of the LastZ alignment of the genomic DNA sequence of two scaffolds. The histogram underneath indicates the local percentage of nucleotide sequence identity of each LastZ High-scoring Segment Pair (HSP). The section in red corresponds to the region shown in panel ( a ). ( c ) Whisker plots (with whiskers representing the range of the distribution, excluding the 5% most extreme values) showing the distribution of percentage of nucleotide sequence identity between LastZ HSPs of 579 ohnologous scaffolds ( n =85,050, red), and the percentage of amino-acid sequence identity between single-copy genes and their pseudogene model ( n =1,344, green) or ohnologous gene copies between each other ( n =4,032, green). Full size image Gene preferentially retained by successive WGDs We analysed the genes originally present in the ancestor of Euteleostomi that were retained in two ohnologous copies after each WGD (1R, 2R, Ts3R, Ss4R). We identified 4,862 ancestral genes retained as 1R or 2R ohnologues in the Human genome, 2,728 ancestral genes retained as Ts3R ohnologues in the zebrafish genome and 4,688 ancestral genes retained as Ss4R ohnologues in the trout genome. The intersection of these three sets of genes ( Fig. 5 ) shows that genes retained as 1R–2R and Ts3R ohnologues are significantly more likely to be retained in duplicated copies after Ss4R ( χ 2 test, P =2 × 10 −16 and 0.03, respectively). The ontology analysis revealed that vertebrate ohnologues are significantly enriched in processes regarding embryonic development and neuronal synapse development and function, and molecular functions involving transcription factors and receptor activity ( Supplementary Table 3 ). However, the gene ontology analysis of the Ss4R ohnologues did not yield any significant results. 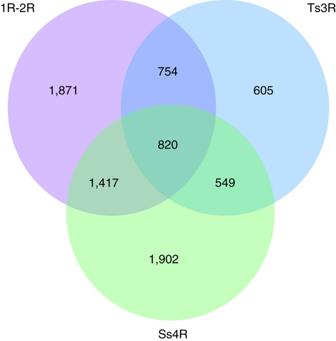Figure 5: Retention of genes as ohnologues after multiple rounds of whole-genome duplication. The gene content of the vertebrate ancestor (Euteleostomi) was reconstructed using Ensembl Compara gene phylogenies. We tested whether genes that were retained as 1R–2R ohnologues in the human genome26, as Ts3R ohnologues in zebrafish7and as Ss4R ohnologues in trout are descended from the same set of ancestral vertebrate genes. We found significant overlaps between the sets, suggesting that some gene families are preferentially retained as ohnologues after WGD events (1R–2R/Ss4R overlap:P=2.10−16; Ts3R/Ss4R overlap:P=0.03;χ2test). Figure 5: Retention of genes as ohnologues after multiple rounds of whole-genome duplication. The gene content of the vertebrate ancestor (Euteleostomi) was reconstructed using Ensembl Compara gene phylogenies. We tested whether genes that were retained as 1R–2R ohnologues in the human genome [26] , as Ts3R ohnologues in zebrafish [7] and as Ss4R ohnologues in trout are descended from the same set of ancestral vertebrate genes. We found significant overlaps between the sets, suggesting that some gene families are preferentially retained as ohnologues after WGD events (1R–2R/Ss4R overlap: P =2.10 −16 ; Ts3R/Ss4R overlap: P =0.03; χ 2 test). Full size image Evolution of gene expression following the Ss4R WGD To better investigate gene fractionation, we carried out an expression analysis across 15 tissues and showed that Ss4R ohnologues still present a remarkable pairwise correlation of their expression profiles ( Fig. 6a and Supplementary Fig. 3 ). However, different clusters of ohnologue pairs displaying specific expression profiles can be identified. Both ohnologues can have statistically correlated expression patterns (high correlation or HC; Pearson’s correlation, P ≤0.05) or not (no correlation or NC; Pearson’s correlation, P >0.05). Additionally, within each group, the two Ss4R ohnologues can present similar average expression levels (similar expression or SE; paired t -test, P >0.05) or one can be consistently overexpressed compared to the other (differential expression or DE; paired t -test, P ≤0.05). These characteristics define four clusters of ohnologues: HCSE, HCDE, NCSE and NCDE ( Fig. 6b ). The pairs of ohnologues in NC clusters present a significantly lower percentage of identity and higher dS, dN and dN/dS compared to the HC clusters (Wilcoxon’s rank sum test, all P <10 −13 ), showing that the divergence of expression patterns is associated with lower selective pressure on the coding sequences ( Fig. 6d and Supplementary Fig. 4 ). Gene ontology analysis reveals that the four types of clusters defined based on expression patterns are clearly associated with different functional classes of genes. The HCSE cluster is enriched in genes involved in development and transcriptional regulation, while the HCDE cluster is enriched in genes involved in housekeeping cellular and metabolic processes. Interestingly, the NCSE cluster, which shows divergent tissue expression between ohnologues, is specifically enriched in genes related to eye development and visual perception ( Fig. 6c and Supplementary Table 4 ) and may correspond to genes for which additional copies can be used as material leading to innovations. 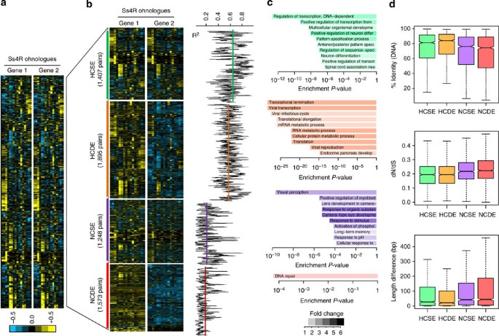Figure 6: Expression of Ss4R ohnologues reveals four classes of genes. (a) Expression levels of ohnologues across 15 tissues (pituitary gland, brain, stomach, white muscle, red muscle, gills, heart, intestine, liver, ovary, bone, skin, spleen, anterior kidney). Expression levels were normalized and centred independently for each Ss4R ohnologue. (b) Delineation of four groups of ohnologues based on (i) correlation between their expression patterns (HC: high correlation,P≤0.05; NC: no correlation,P>0.05; Pearson’s correlation test), and (ii) their relative expression levels (SE: same expression levels,P>0.05; DE: different expression levels,P≤0.05; Student’s pairedt-test). Expression levels were normalized and centred across both ohnologues in the left panel, highlighting differences in relative levels of expression between both genes. Pearson’s correlation coefficients between the expression levels of both ohnologues across all tissues are represented in the right panel. (c) Top functional enrichments for each class of ohnologues, compared with the remainder of the ohnologue set. Each class of ohnologues corresponds to a functionally distinct group of genes. EnrichmentP-values were obtained using Fisher’s exact test; colours highlight the fold change between expected and observed genes annotated with a given ontological term (Supplementary Table 3for the complete list of enriched terms and methodological details). (d) Whisker plots (with whiskers representing the range of the distribution, excluding the 5% most extreme values) showing the sequence conservation for each class of ohnologues (numbers of ohnologue pairs HCSE=1,407; HCDE=1,895; NCSE=1,248; NCDE=1,573). Highly correlated ohnologues are on average significantly more conserved at the sequence level and under higher selective pressure (as described by dN/dS ratios) than non-correlated ohnologues, showing that divergence in expression patterns is associated with divergence of the coding sequence. Figure 6: Expression of Ss4R ohnologues reveals four classes of genes. ( a ) Expression levels of ohnologues across 15 tissues (pituitary gland, brain, stomach, white muscle, red muscle, gills, heart, intestine, liver, ovary, bone, skin, spleen, anterior kidney). Expression levels were normalized and centred independently for each Ss4R ohnologue. ( b ) Delineation of four groups of ohnologues based on (i) correlation between their expression patterns (HC: high correlation, P ≤0.05; NC: no correlation, P >0.05; Pearson’s correlation test), and (ii) their relative expression levels (SE: same expression levels, P >0.05; DE: different expression levels, P ≤0.05; Student’s paired t -test). Expression levels were normalized and centred across both ohnologues in the left panel, highlighting differences in relative levels of expression between both genes. Pearson’s correlation coefficients between the expression levels of both ohnologues across all tissues are represented in the right panel. ( c ) Top functional enrichments for each class of ohnologues, compared with the remainder of the ohnologue set. Each class of ohnologues corresponds to a functionally distinct group of genes. Enrichment P -values were obtained using Fisher’s exact test; colours highlight the fold change between expected and observed genes annotated with a given ontological term ( Supplementary Table 3 for the complete list of enriched terms and methodological details). ( d ) Whisker plots (with whiskers representing the range of the distribution, excluding the 5% most extreme values) showing the sequence conservation for each class of ohnologues (numbers of ohnologue pairs HCSE=1,407; HCDE=1,895; NCSE=1,248; NCDE=1,573). Highly correlated ohnologues are on average significantly more conserved at the sequence level and under higher selective pressure (as described by dN/dS ratios) than non-correlated ohnologues, showing that divergence in expression patterns is associated with divergence of the coding sequence. Full size image Genome evolution following WGD is thought to involve the loss of one gene copy of most ohnologous gene pairs by a process termed gene fractionation [10] . The early steps of this process have never been documented at the whole-genome scale in vertebrates because all WGDs studied to date are too ancient [2] , [8] , [9] to allow such analysis. The rainbow trout genome sequence provides, for the very first time in any vertebrate, a unique opportunity to build a possible scenario on these early steps of gene fractionation occurring after a WGD event. We first use the rainbow trout genome to refine the timing of the Ss4R and we dated this event around 96 Mya (±5.5 Mya), a timing in the upper range of the previous 25–100 Mya estimation [11] . This result is in striking contrast with the age of the Salmonidae family, which has been estimated as 50–60 Mya [4] , [16] , suggesting that the Ss4R occurred long before the last common ancestor of extant salmonids. This observation is consistent with the WGD Radiation Lag-Time Model [17] that has been proposed in plants in which significant lag times would be needed between WGDs and the subsequent adaptive radiations that are often associated with these WGD events [17] , [18] . Despite this 100 My of evolution since the Ss4R, we found many evidences of an extreme stability of the two ancestral genome copies in the rainbow trout genome. At the chromosome level, no pervasive rearrangements were observed, and the structure of the Ss4R paralogous sequences remains surprisingly well conserved in sequence identity and gene order on chromosomes. Together these observations show that gene fractionation does not involve many genomic rearrangements such as inversions or translocations that would modify the order of genes in the genome, or large deletions that would result in long clusters of singletons. At the gene level we estimated the number of genes in the pre-Ss4R salmonid ancestor to be ∼ 31,000 genes. Interestingly, the zebrafish genome, the teleost fish with the most exhaustive and well-supported protein-coding gene annotation to date, contains ∼ 26,000 genes. This figure of 31,000 genes estimated here for the ancestral salmonid genome is compatible with the modern estimate in zebrafish, since, being 100 My closer to the event, the pre-Ss4R ancestral salmonid was likely to contain more duplicated gene copies remaining from the teleost Ts3R WGD. After 100 My of evolution since the Ss4R, gene fractionation only affected half of the ancestral Ss4R ohnologues, which have now returned to a single-copy state, resulting in an average gene inactivation rate of ∼ 170 genes per My. In contrast with the idea that gene fractionation after WGD involves massive and rapid gene deletions, we found numerous traces of pseudogenization events, and most of these pseudogenes exhibit a low sequence divergence compared to their respective functional copy. These numerous pseudogenization events may have initiated subsequent deletions that we also observe, and thus played a major role in the rediploidization of the trout genome. Altogether these multiple evidences suggest that gene fractionation is a slow process, largely incomplete and still in progress in the trout genome. This challenges the current hypothesis that WGDs are followed by massive and rapid genomic reorganizations and gene deletions [19] , [20] . In plants, it has been suggested that preferential retention of singletons is localized on one of the two chromosomes from the WGD, leading to the appearance of a ‘dominant’ chromosome in the modern genome [21] . The distribution of the ohnologues on the duplicated chromosomes of rainbow trout does not support such a hypothesis in vertebrates. In striking contrast with the retention of half of the protein-coding genes as ohnologues is the nearly complete retention of miRNA gene as duplicate copies originating from the Ss4R. Together with the differences in the number of loci per mature miRNA observed in trout, and to a lower extent in teleost, in comparison with tetrapods and non-vertebrate metazoans, these results indicate that the fractionation process is considerably slower for miRNA genes than for protein-coding genes. This difference is unlikely to be explained by the short sequence of miRNA genes ( Supplementary Note 1 ). It is, however, noteworthy that miRNAs are acting in a dose-dependent manner to tune gene expression at post-transcriptional level [22] and that miRNAs have several, if not many, targets among protein-coding mRNAs [23] . It is thus possible that all duplicated copies of miRNA genes are still necessary to control gene expression in the context of a recent WGD. The fractionation process of miRNA genes would then occur, in a second step, at the end of the protein-coding gene fractionation process. Our analysis also revealed that genes retained in duplicated copies after the successive WGD events that occurred during vertebrate evolution were also more likely to be retained as duplicates following Ss4R. This observation confirms the preferential retention and amplification of a number of gene families over successive WGD events [7] , [24] , [25] . Our results show that genes preferentially retained by successive WGDs are associated with specific ontologies, in consistency with several studies that have shown preferential retention of some functional categories of genes among ohnologues present in modern vertebrate genomes [26] , [27] . However, the gene ontology analysis of Ss4R ohnologue did not yield significant results, possibly because gene fractionation is still largely in progress and the set of trout ohnologues has not yet narrowed down to genes selectively retained as duplicates. Finally, while the conservation of the structure and expression of the two ancestral genome copies is remarkable, a substantial number of Ss4R ohnologues have strongly diverged in terms of expression profiles and/or expression levels. Following WGDs, it is well accepted that the remaining ohnologues can acquire new expression patterns potentially leading to neo- or subfunctionalization [28] . This suggests that evolution after WGD is also acting on regulatory regions of these ohnologous genes that could subsequently be either silenced, or sub- or neo-functionalized. Together, the analysis of the rainbow trout genome reveals a slow and stepwise rediploidization process after the Ss4R that challenges the current hypothesis that WGD is followed by massive and rapid genomic reorganizations and gene deletions. Genome sequencing The 454 (single read, and 8-, 12- and 20-kb mate pairs) genomic libraries were prepared following the manufacturer’s protocol (GS FLX Titanium Library Preparation Kit, Roche Diagnostic, USA) using genomic DNA from a single homozygous doubled haploid YY male from the Swanson River (Alaska) clonal line [29] , [30] ( Supplementary Methods ). Libraries were quantified and evaluated using a 2100 bioanalyzer (Agilent Technologies, USA). Each library was sequenced using Pico Titer Plates on a 454 GSFlx instrument with Titanium or long read chemistry (Roche Diagnostic, USA). Genomic Illumina libraries were constructed according to the Illumina standard procedure for shearing of genomic DNA, end repair and adaptor ligation. The enrichment PCR was performed using Platinum Pfx DNA polymerase (Invitrogen). Amplified library fragments were size-selected to 300–600 bp on a 3% agarose gel. Each library was sequenced using 76 or 100 base-length read chemistry in paired-end and single-read flow cells on the Illumina GA IIx/HiSeq2000 (Illumina, USA). Genome assembly Public Sanger BAC-end sequences (BES) [31] and Roche/454 reads ( Supplementary Table 5 ) were assembled together with Newbler (version MapAsmResearch-04/19/2010-patch-08/17/2010). The total size of the resulting assembly was 1.9 Gb with a scaffold N50 of 384 kb (half of the assembly is contained in 1,014 scaffolds longer than 384 kb, Supplementary Table 6 ). Sequence quality of scaffolds from the Newbler assembly was improved by automatic error corrections with Solexa/Illumina reads [32] (70-fold genome coverage), which have a different bias in error type compared to 454 reads ( Supplementary Methods ). The genome sequence and annotation can be obtained and viewed at https://www.genoscope.cns.fr/trout/ Genome annotation Repeated regions of the assembly (37.8%) were masked against: (i) a collection of 634 motifs that we characterized using RepeatMasker ( http://www.repeatmasker.org ), (ii) low complexity sequences using DUST [33] , (iii) tandem repeats using Tandem Repeat Finder [34] , (iv) teleost repeats from RepBase [35] , and (v) simple repeats using Repeat Masker. In addition, we integrated predictions of repeated motif from RepeatScout [36] in the final gene prediction models ( Supplementary Methods ). To refine exon/intron junction locations, 305,000 teleost protein sequences from Uniprot [37] and Ensembl [38] were aligned on the genome sequence using the BLAT algorithm [39] to first select the best match (plus matches greater than 0.8X best matches) and each matched protein was then realigned using Genewise [40] on the same trout genomic region. 93% of these teleost proteins matched at 41,300 different genomic loci in the rainbow trout genome assembly. For building gene models, rainbow trout GenBank mRNA sequences were aligned onto the genome assembly using BLAT [39] and est2genome [41] resulting in 93% of mapping of these 421,414 mRNA sequences. Only the best matches with at least 90% of nucleotide identity were kept. On average, similarity level was 97.8% and half of these alignments supported splicing evidence, with an average of 2.5 exons per mRNA. We also used publicly available rainbow trout Roche 454 EST sequences available in SRA (accession number SRX007396 ) that were assembled using Newbler, and aligned using blat and est2genome with the same setting used for mRNAs. A total of 97% of these cDNA contigs were mapped on the rainbow trout assembly at 45,600 different genomic loci. In addition, we generated Illumina reads of different tissue transcriptomes (see below) that were also used to predict exon/intron structure on the genome assembly using gMorse [42] . Using all these resources we predicted 69,676 transcripts with an average size of 4.8 Kb (median size of 2.1 Kb), and an average exon number of 6.7 (median=4). Overall, 7.7% of the assembly is targeted by a transcriptional signal. Final gene models were built using Gaze [43] leading to 55,735 gene models with an average of 6 exons per gene (median=4). At the genome level, coding bases cover 3% of the assembly. Because 3,088 exons were overlapping gaps in the assembly, we inserted in-frame introns to avoid a long stretch of N letters in the corresponding protein sequences. We also tagged 585 genes that still contained transposable elements despite repeated cleaning procedures. In summary, the final gene set can be categorized into 4 classes of decreasing confidence level: (i) 46,585 protein-coding gene models with supporting protein evidence from other vertebrates ( Supplementary Table 7 ), (ii) 6,789 genes lacking protein evidence without any assembly gap and with a transcriptional signal deduced from cDNA, (iii) 1,451 genes lacking protein evidence, without any assembly gap, and without a transcriptional signal deduced from cDNA, and (iv) 890 genes lacking protein evidence which overlap assembly gaps. Sequence anchoring using genetic and physical maps Correspondence between linkage groups and chromosomes was done according to Phillips et al. [44] A sequential use of data from linkage and physical maps was applied to anchor the sequence assembly to chromosomes. The first anchoring step was performed using markers from a consensus linkage map [14] . The sequence assignment was then expanded using BES information from the trout physical map [45] , [46] , [47] , and markers from a RAD based linkage map [48] . Using this linkage and physical map information, 4,413 sequences were assigned to 898 distinct loci on the genetic map and locally ordered representing a total sequence length of 1,023,288,475 bp, that is, 48% of the total assembly, and 54% of total length of the scaffolds ( Supplementary Table 8 and Supplementary Methods ). Rainbow trout transposable elements Annotation of transposable elements was done using BES of O. mykiss and Salmo salar , 60 completely sequenced rainbow trout BAC, cDNA Unigene library and the rainbow trout genome sequence. Classification of TEs was based on Wicker’s classification [49] . A database of TEs was built combining both manual and automatic annotation ( Supplementary Methods ). Transposable elements account for ∼ 38% of the rainbow trout genome sequence ( Supplementary Table 9 ). To evaluate the age of TE copies, Kimura distances were calculated based on the alignment (consensus from the TE library versus copy in the genome) generated by RepeatMasker. The Kimura calculation uses the rates of transitions and transversions. Those rates are then transformed in Kimura distances using the formula K =−1/2 ln(1–2 p – q )–1/4 ln(1–2 q ), where ‘ p ’ is the proportion of site with transitions and ‘ q ’ the proportion of site with transversions. Using Kimura distances, we estimated the relative age of the different TE families in the genome of the rainbow trout ( Supplementary Fig. 5 ). It appears that two or three main bursts of transposition occurred in the genome. The most ancient one is mainly due to a high activity of Tc-Mariner families (Kimura value 41). In the second (around Kimura value 12), an increase of all families and particularly CR1 is highlighted. Finally, the last one (Kimura value 8) shows a new burst of Tc-Mariner activity. Rainbow trout WGDs and comparative genome analyses As a starting point for comparative genome analyses, we integrated predicted trout genes in vertebrate gene families based on Ensembl version 66 (February 2012) [50] . The 46,585 predicted trout proteins were compared against 13,264 gene families from 14 representative vertebrate species comprising mammals, birds and fish ( Supplementary Fig. 6 ). Trout genes were included in 8,739 vertebrate gene trees ( Supplementary Table 7 ). By comparison, other genes from other vertebrate genomes are included in 7,131 (takifugu) to 9,453 (Human) gene families, suggesting that annotated trout genes cover the vast majority of vertebrate gene families. A dedicated Genomicus server ( http://www.genomicus.biologie.ens.fr/genomicus-trout-01.01/ ) provides access to trout genes and their phylogenetic trees, as well as syntenic relationships with other genomes ( Supplementary Fig. 7 ). DCS blocks are defined as runs of genes in a non-salmonid (that is, non-duplicated by the Ss4R event) genome that are distributed on two different chromosomes (or non-anchored scaffolds) in the rainbow trout genome; the exact gene order does not need to be conserved. We systematically compared the gene locations in rainbow trout with those of medaka, stickleback, tetraodon and takifugu using ad-hoc scripts to identify pairs of regions in the rainbow trout genome that are syntenic with single regions in non-salmonid species, and that correspond to DCS blocks. Pairs of paralogous trout genes on two different chromosomes (or non-anchored scaffolds) that belong to a DCS block are most likely duplicates originating from the Ss4R WGD event and are called ohnologues; there were 6,733 pairs of ohnologues. Genes that are inserted in a DCS block based on synteny with a non-salmonid species, but have no paralogous gene on the other chromosome or scaffold, are most likely former Ss4R duplicates in which one of the duplicated genes was lost, and are called singletons. Each pair of duplicated regions within a DCS block is descended from a single ancestral region in the pre-duplication genome. The organization of these ancestral regions into an ancestral chromosome was deduced from the synteny relationships with non-salmonid genomes using a clustering method implemented in Walktrap [51] . The Ts3R-duplicated regions in the ancestral karyotype were obtained by orthology with the Ts3R-duplicated regions in the medaka genome, which were themselves deduced from the DCS blocks between the medaka and chicken genomes obtained as described above. DCS blocks can be very short, as they are dependent on assembly continuity and scaffold anchoring. Fine-scale analysis of duplicated regions and genes was restricted to 915 scaffolds that could be paired into 569 DCS blocks for at least part of their lengths, and that share at least 4 ohnologous genes. The longest scaffold in these DCS blocks is 5,466,130 bp long and the shortest is 25,207 bp long. These 915 scaffolds contain a total of 171 miRNAs and 13,352 genes (29% of the trout genome), of which 8,624 are ohnologues and 4,728 are singletons. These scaffolds were aligned using LastZ [52] , resulting in 85,050 local alignments with a mean identity of 86.7%. To better understand the fate of inactivated gene copies, protein sequences predicted from a given gene model were also aligned to their paralogous region using exonerate [53] with the ‘—model protein2genome’ option ( Supplementary Methods ). Rates of gene loss since the Ts3R WGD were calculated by linear extrapolation. Rates of molecular evolution Atlantic salmon ( S. salar ) coding mRNA sequences (12,062 sequences) [54] were translated into protein sequences. Blastp reciprocal best hits between these salmon and trout proteins were aligned with MUSCLE [55] , [56] , and rates of silent substitution (dS values) of the corresponding coding sequences were calculated using the Yang and Nielsen method in PAML4.4 (ref. 57 ). Ohnologous gene sequences from fish genomes were obtained from Ensembl Treebest gene trees and DCS analyses. MUSCLE alignment of protein sequences followed by PAML4 analysis of the coding sequences (CDS) was used to compute the dS and dN values for pairs of ohnologous sequences originating from the Ts3R WGD in stickleback, tetraodon, medaka and zebrafish, and for trout Ss4R ohnologues. Trout Ts3R ohnologues represent a special case, because each copy (for example, A and B) was further duplicated by the Ss4R, and thus may be represented by one (if the other Ss4R ohnologue was lost) or two sequences (for example, A1, A2 and B1, B2). A given Ss4R ohnologue was always aligned separately to each Ss4R duplicate copy stemming from the Ts3R (for example, A1 to B1 and B2), when they existed. Alignments were then concatenated to compute dS values, which thus represents an average dS (resp. dN) value for the Ts3R duplication for a given family of ohnologues. When Ss4R ohnologues existed in more than two copies, because of subsequent local duplication (for example, A1, A2, A3), we aligned each possible combination of pairs using MUSCLE [55] , [56] (for example, A1–B1, A2–B1, A3–B1, etc.) and then concatenated alignments as before (for example, A1–B1 with A2–B1), in all possible combinations of two concatenated alignments, each leading to a dS (resp. dN) value. The smallest dS value among all alignments was considered the most conservative and retained for further analysis, together with the corresponding dN. The rate of selective constraints on orthologues and ohnologues was calculated with PAML4.4 ( ω =dN/dS) using the method of Yang and Nielsen [58] . A linear extrapolation from the dS comparison was used to infer the timing of the Ss4R. Transcriptome sequencing and data analysis Tissues for transcriptome analyses were obtained from a homozygous clonal 1-year-old female sampled 3 weeks after spawning. These doubled haploid females were first produced after gynogenetic reproduction of standard females plus inhibition of first embryonic cleavage [59] , and further reproduced by a second round of gynogenesis (inhibition of second meiosis) [60] . Homozygous clonal lines were further maintained during every generation by single within-line pair mating between one female and one hormonally sex-reversed male. Tissues (liver, brain, heart, skin, ovary, white and red muscle, anterior and posterior kidney, pituitary gland, stomach, gills) were collected and stored in liquid nitrogen until RNA extraction. Total RNA was extracted using Tri-reagent (Sigma, St-Louis, USA) at a ratio of 100 mg of tissue per ml of reagent according to the manufacturer’s instructions. RNA-Seq Illumina Libraries were prepared ( Supplementary Methods ) and sequenced using 101 base-lengths read chemistry on an Illumina GAIIx sequencer (Illumina, USA). In order to compare the expression levels of ohnologous genes, we restricted the analysis to the parts of the coding regions that can be confidently aligned using MUSCLE [56] between the two genes, as non-alignable or low-quality alignment regions may result from errors in the automatic annotation process. We retained regions of the alignment where the majority of codons contain at most 1 nucleotide change, and masked all other codons with Ns. We mapped RNA-seq reads to these alignable regions using BWA [61] with stringent mapping parameters (maximum number of mismatches allowed –aln 2). Mapped reads were counted using SAMtools [62] , with a minimum alignment quality value (–q 30) to discard ambiguous mapping reads. The numbers of mapped reads were then normalized for each gene across all tissues using DESeq [63] . As the alignable regions of both ohnologues are of the same length by construction, no additional normalization for length was necessary to compare expression levels within each ohnologue pair. Correlations between the expression levels of ohnologues were performed using Pearson’s correlation and paired Student’s t -tests in R on log2-transformed data. Log2-transformed expression profiles of rainbow Ss4R ohnologues were also analysed using supervised clustering methods. Hierarchical clustering was processed using centroid linkage clustering with Pearson’s uncentred correlation as similarity metric on data that were normalized and median-centred using the Cluster program [64] . Expression levels were normalized and centred independently for each Ss4R ohnologue pair to compare expression profiles ( Fig. 4a ) and normalized and centred across both ohnologues to highlight differences in relative levels of expression between both ohnologous genes ( Fig. 4b ). Results (colorized matrix) of hierarchical clustering analyses were visualized using the Java TreeView program [65] . miRnome sequencing and data analysis miRNA sequencing was performed from several adult tissues (brain, muscle, gills, intestine, heart, liver, pituitary, skin, leucocytes, kidney, reproductive tissue, intestine, stomach and spleen) and whole embryos (NCBI BioProject ID No. PRJNA227065). Total RNA was extracted as described for transcriptome sequencing. Because of the high egg yolk content of vitellogenic ovaries, ovarian samples were subsequently purified using a NucleoSpin miRNA kit (Macherey Nagel, Germany). RNA integrity was checked using an RNA 6000 Nano chip (Agilent). Small RNA libraries were constructed according to the Illumina Small RNA v1.5 sample preparation guide ( Supplementary Methods ) and were sequenced with a 36-bp chemistry on an Illumina HiSeq-2000 sequencer. A total of 3,484,155,614 reads were generated from the 38 sequenced libraries. Low-quality sequences were filtered and adaptors removed from raw small RNA sequence data using the FastQC and Cutadapt programs [66] , respectively. Intra- and inter-condition redundancy was eliminated and annotations of known miRNAs were performed as follows: reads were blasted to miRBase database [67] , Rfam database [68] , rRNA-silva database [69] and tRNA database [70] . Reads with hits in miRBase and Rfam but not in rRNA or tRNA database were kept as potential miRNAs. We only kept reads with more than 1,000 hits (among all conditions) to build strong loci. Reads were subsequently aligned to the trout genome with the following filters: exact match or maximum 95% suboptimal best hit with a maximum of 15 localizations within the genome sequence. miRNA-5p/miRNA-3p loci were built as follows: sequences belong to the same locus if there is no base difference among sequences and if miRNA-5p and miRNA-3p are at least 30 nucleotides distant from each other. This allowed the identification of 495 miRNA loci corresponding to 84 different families and 164 mature sequences ( Supplementary Data 1 ). Gene ontology analyses GO analyses were performed in two steps. Statistically enriched functional annotations were obtained in the sample set using a random sampling procedure (10,000 iterations, custom Perl script) with corrected false discovery rate for multiple testing (Benjamini–Hochberg FDR correction, with a 10% FDR threshold). The exact enrichment P -values for GO terms detected as significant through the random sampling procedure were then calculated using Fisher’s exact test in R ( Supplementary Methods ). Accession codes : Genome, transcriptome and miRNA sequence data for Oncorhynchus mykiss have been deposited in GenBank/EMBL/DDBJ sequence read archive (SRA) under the accession codes ERP003734 , ERP003742 and SRP032774 . The genome assembly has been deposited in the European Nucleotide Archive under the accession code CCAF000000000 and the project PRJEB4421. How to cite this article: Berthelot, C. et al. The rainbow trout genome provides novel insights into evolution after whole-genome duplication in vertebrates. Nat. Commun. 5:3657 doi: 10.1038/ncomms4657 (2014).